Gains to species diversity in organically farmed fields are not propagated at the farm level Organic farming is promoted to reduce environmental impacts of agriculture, but surprisingly little is known about its effects at the farm level, the primary unit of decision making. Here we report the effects of organic farming on species diversity at the field, farm and regional levels by sampling plants, earthworms, spiders and bees in 1470 fields of 205 randomly selected organic and nonorganic farms in twelve European and African regions. Species richness is, on average, 10.5% higher in organic than nonorganic production fields, with highest gains in intensive arable fields (around +45%). Gains to species richness are partly caused by higher organism abundance and are common in plants and bees but intermittent in earthworms and spiders. Average gains are marginal +4.6% at the farm and +3.1% at the regional level, even in intensive arable regions. Additional, targeted measures are therefore needed to fulfil the commitment of organic farming to benefit farmland biodiversity. Biodiversity is threatened, both at global and regional scales [1] , [2] . During the past decades, agriculture has been a key driver of the loss of biodiversity through intensification of existing farmland and conversion of natural land into cropland [3] , [4] , [5] . However, farmland also hosts many species that depend on appropriate agricultural management for their survival [6] , [7] . Organic agriculture is intended to be a biodiversity-friendly and sustainable farming system [8] and is promoted by many countries as a way of reducing the environmental impacts of agriculture [9] . Although debated, better food quality [10] and less environmental impact [11] are persuasive arguments that have encouraged an increasing number of consumers to buy organic products. Organic farming is also considered a key strategy for land sharing, that is, the promotion of biodiversity and food production on the same area of land [5] , [12] , [13] , [14] . Evidence generally suggests that organic farming has beneficial effects on biodiversity, but the magnitude of these effects is highly variable [11] , [15] , [16] , [17] , [18] , [19] , [20] , [21] , [22] . This is due to two major challenges in quantifying the effects of a farming system on biodiversity. First, biodiversity is prohibitively expensive to capture comprehensively and therefore only inferable using proxies, for example, species richness of certain ‘indicator’ taxonomic groups [23] , [24] . A meta-analysis indicated that organic farming increases species evenness and that organic farming gains to species richness are mainly effects of the abundance of individuals [25] . The second challenge is that, while research investigates biodiversity mostly at the field scale, a farmer considers his entire farm when making management decisions [26] . Farms are highly diverse in their internal organization and spatial layout, even within the same geographical region and production type. Farming effects at the field level do not necessarily translate directly to the farm or landscape level [12] , [15] , [18] , [19] , [27] . Hence, studies at multiple scales are crucial to understanding the impacts of farming systems on biodiversity [28] . In a large study on farmland biodiversity, we aimed to quantify the benefits organic farming has on species diversity at field, farm and regional levels across a range of environments from boreal to tropical. To address the challenge of the intangible nature of ‘biodiversity’ as a whole, we analysed organism abundance, species richness and species evenness in four taxonomic groups: plants, earthworms, spiders and bees. The groups were selected to represent different habitat compartments (soil, soil surface and above-ground structures), trophic levels, mobility and expected responses to agricultural management [15] , [16] , [19] , [20] , [29] , [30] . To cope with the heterogeneity of agriculture, we sampled species in 205 farms in twelve contrasting regions in Europe and Africa using standardized methods ( Fig. 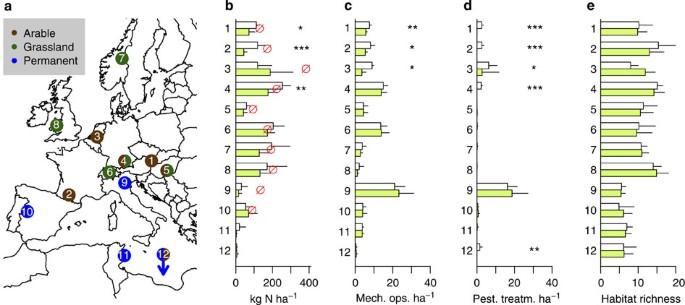Figure 1: Management of organic and nonorganic farms in twelve regions on two continents. (a) Location of study regions with predominant type of agricultural land use and country boundaries62. Regions with bicolour symbol have mixed land use (seeTable 1for details). Region 12 is located in Uganda and not shown on map. (b–d) Average nitrogen input per hectare (+s.d.) (b), average number of mechanical operations (c), average number of pesticide applications (d) and average number of habitats (e) in nonorganic (white bars) and organic farms (green bars) in the twelve regions. Red Ø are national average N inputs in 2008 (ref. 43)43. Significant differences within regions (U-test) at 0.05, 0.01 and 0.001 are indicated by *, ** and ***, respectively. mech. ops., mechanical operations; pest. treatm., pesticide treatment. 1a ; Table 1 ). The regions were homogeneous with regard to environmental conditions, and from each region, 12 to 20 farms were randomly selected, approximately half of them certified organic. No additional constraints were set on the nonorganic farms, which could therefore comply with various other statutory or voluntary standards of environmental care [31] . This provided us with representative samples of present-day organic and nonorganic farms of a particular production type in every region, thereby avoiding the problematic, and ultimately impossible, exercise of pairing organic and nonorganic farms. The consistent assessment of species diversity across three levels of aggregation identifies decreasing gains to species diversity from field to farm and region and recommends targeted measures for the promotion of farmland biodiversity. Figure 1: Management of organic and nonorganic farms in twelve regions on two continents. ( a ) Location of study regions with predominant type of agricultural land use and country boundaries [62] . Regions with bicolour symbol have mixed land use (see Table 1 for details). Region 12 is located in Uganda and not shown on map. ( b – d ) Average nitrogen input per hectare (+s.d.) ( b ), average number of mechanical operations ( c ), average number of pesticide applications ( d ) and average number of habitats ( e ) in nonorganic (white bars) and organic farms (green bars) in the twelve regions. Red Ø are national average N inputs in 2008 (ref. 43) [43] . Significant differences within regions ( U -test) at 0.05, 0.01 and 0.001 are indicated by *, ** and ***, respectively. mech. ops., mechanical operations; pest. treatm., pesticide treatment. Full size image Table 1 Locations and environmental characteristics of the study regions. Full size table Farm structures and management The investigated regions represented various production types with a low-to-medium intensity of farming, thus accounting for a relatively large portion of global agriculture [32] . Regional average nitrogen (N) input ranged from 5 to 215 kg N ha −1 ( Fig. 1b ), average farm sizes per region were between 3 and 142 ha ( Supplementary Table 1 ). Organic farms were characterized by lower mean nitrogen inputs (−22.4%, <0.02; Fig. 1b ), fewer mechanical field operations (−9.3%, <0.08; Fig. 1c ), and fewer pesticide applications (−75.9%, <0.001; Fig. 1d ) than in their nonorganic counterparts. Organic farms did not, on average, have a higher number of habitat types or a higher areal proportion of semi-natural elements ( Fig. 1e ). Species richness in production and nonproduction habitats As habitats present in each region differed, a comparison at the field level was only possible for the most frequently observed habitats per study region. 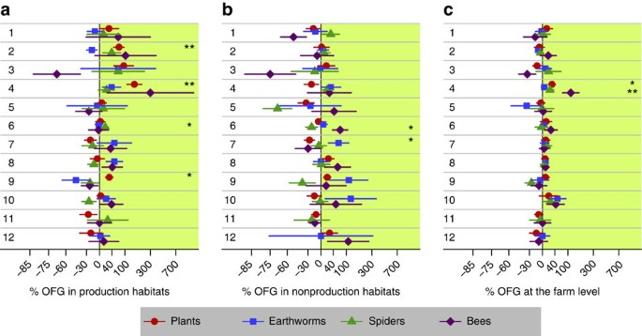Figure 2: Organic farming gains and losses to species richness in twelve regions. Organic farming gains/losses (OFG, ±s.d.) to species richness in the regionally most frequent production habitats (a), in the most frequent nonproduction habitats (b) and on total species richness per farm (c), for the four taxonomic groups of plants, earthworms, spiders and bees in the twelve regions shown inFig. 1a.Xaxes are log-scaled to equalize distances on both sides of parity. Significant differences within regions (U-test) at 0.05 and 0.01 are indicated by * and **, respectively. Depending on the region, the most frequent habitats managed with the primary aim of agricultural production were winter or summer-sown non-entomophilic crop fields, fertile grasslands, vineyards or olive groves ( Supplementary Table 2 ). The most frequent nonproduction habitats, for example, managed for access to land, wind shelter or as part of an agri-environmental scheme, were grassy or shrubby strips along field or water edges. Organic farming was beneficial to species richness of plants and bees in production fields in many regions, but differences were rarely significant if tested within each region separately ( Fig. 2a ). Mixed-effects models estimated by maximum likelihood show that in all regions combined, organic farming gains to species richness in production habitats were +17.1% ( <0.01) for plants, +6.3% (NS) for earthworms, +1.2% (NS) for spiders, +13.6% (NS) for bees. Across all four taxonomic groups and all regions, 10.5% ( <0.02) more species were found in organic than in nonorganic production fields. This significant positive effect of organic farming on species richness arises from the fact that all groups responded positively, although only the difference in plants was significant. Figure 2: Organic farming gains and losses to species richness in twelve regions. Organic farming gains/losses (OFG, ±s.d.) to species richness in the regionally most frequent production habitats ( a ), in the most frequent nonproduction habitats ( b ) and on total species richness per farm ( c ), for the four taxonomic groups of plants, earthworms, spiders and bees in the twelve regions shown in Fig. 1a . X axes are log-scaled to equalize distances on both sides of parity. Significant differences within regions ( U -test) at 0.05 and 0.01 are indicated by * and **, respectively. Full size image Differences in species richness between organic and nonorganic production fields were highest in winter-sown crops in Marchfeld, Gascony and Southern Bavaria as well as in the horticultural fields in Gelderland (+45.5%, <0.001 on average across these four regions and the four taxonomic groups). Effects were similar if the regionally most frequent individual crops (winter wheat or alfalfa) were compared ( Supplementary Fig. 1 ). These crops were not necessarily present on all farms because details of the crop rotation were not a selection criteria but rather a possible difference between farms. The four regions also showed significant differences in management intensity between organic and nonorganic farms (as illustrated by N input, the number of mechanical operation per ha and the number of pesticide applications per ha; Fig. 1b–d ). Average regional gains to species richness in production habitats were positively correlated to regional average N input per ha (Spearman’s ρ =0.68, P <0.05). In contrast to production habitats, organic farming did not alter species richness in nonproduction habitats (−3.6% (NS) for plants, +13.4% (NS) for earthworms, −7.1% (NS) for spiders, +9.1% (NS) for bees and −0.7% (NS) overall; Fig. 2b ). Organic farming gains to species richness at the farm level As assessed by hierarchical preferential sampling, organic farms tended to have higher total species richness than nonorganic farms. Across all regions, organic farming gains were +4.8% (NS) for plants, +3.1% (NS) for earthworms, +3.2% (NS) for spiders, +12.8% ( < 0.05) for bees and +4.6% ( <0.1) across all four taxonomic groups. Gains to total species richness were strongest in Bavarian mixed farms, as well as in olive farms in Extremadura, and were consistently positive in the grassland farms in Obwalden, Hedmark and Wales ( Fig. 2c ). These results reflect diminished organic farming gains for biodiversity when observed at the farm level as compared with the field level. A weighted random resampling procedure with the areal proportion of different habitats per farm as weights indicated that organic farming gains to species richness decrease if more of the smaller habitats on the farm are included ( Fig. 3a–d ). The resampling mimicked random species sampling, in which samples are more likely drawn in habitats with a larger areal proportion, in this case, predominantly production habitats. The fading was especially pronounced where organic farming gains to production habitats were large, namely with plants and bees and in regions with arable cropping ( Fig. 3e ). Gains to species richness of spiders also tended to decrease with more sampled habitats. 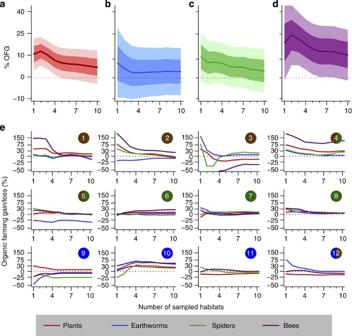Figure 3: Organic farming gains and losses to species richness fade from field to farm. (a–d) Species numbers of plants (a), earthworms (b), spiders (c) and bees (d) depending on the number of resampled habitats in the twelve regions shown inFig. 1a. Lines show average organic farming gains/losses (OFG) estimated from mixed-effects models, shaded areas are approximate 50 and 95% confidence intervals. (e) Species numbers depending on the number of resampled habitats for the twelve individual regions.Yaxes are log-scaled to equalize distances on both sides of parity. Numbers and coloured circles correspond to the twelve regions as displayed inFig. 1a. Figure 3: Organic farming gains and losses to species richness fade from field to farm. ( a – d ) Species numbers of plants ( a ), earthworms ( b ), spiders ( c ) and bees ( d ) depending on the number of resampled habitats in the twelve regions shown in Fig. 1a . Lines show average organic farming gains/losses (OFG) estimated from mixed-effects models, shaded areas are approximate 50 and 95% confidence intervals. ( e ) Species numbers depending on the number of resampled habitats for the twelve individual regions. Y axes are log-scaled to equalize distances on both sides of parity. Numbers and coloured circles correspond to the twelve regions as displayed in Fig. 1a . Full size image Effects of organic farming on organism abundance and species evenness Organic farming gains to organism abundance and to species richness were strongly correlated (Spearman’s ρ =0.67, P <0.001, over all four groups in production and nonproduction habitats and at farm level; Supplementary Table 3 ). Consequently, trends for organic farming gains were also detected for the cumulated cover abundance of plants (+9.0%, NS) and the number of individuals of earthworms (+3.8, NS), spiders (+5.7%, NS) and bees (+23.8, NS) in production habitats ( Fig. 4a ). As with species richness, organic farming gains to organism abundance across all four taxonomic groups were highest for the four regions with intensive arable or horticultural fields (+25.6%, <0.05 versus +8.5%, NS, across all regions). Rarefying faunal species richness to equal numbers of sampled individuals showed that a positive but insignificant gain of organic farming remained (+6.9%, NS, for earthworms; +2.0% for spiders and +9.8% for bees; Supplementary Fig. 2 ). Organic farming had no significant effect on species evenness in production habitats, with the exception of plants in the four most intensive regions (+40%, <0.01; Supplementary Fig. 3 ). Organic farming also had no significant effects on abundance or evenness in nonproduction habitats ( Fig. 4b and Supplementary Fig. 3 ) and at the farm level ( Fig. 4c and Supplementary Fig. 3 ). 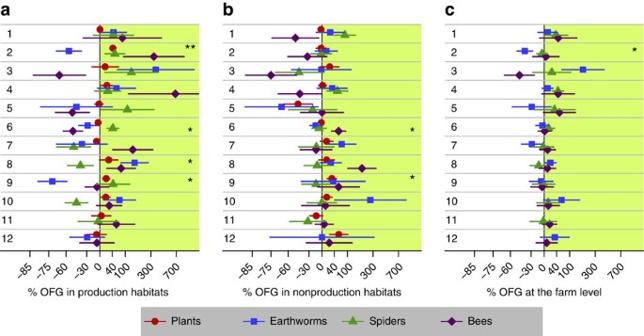Figure 4: Organic farming gains and losses to organism abundance in twelve regions. Organic farming gains/losses (OFG, ±s.d.) to organism abundance for the four taxonomic groups (cumulated cover for plants and number of individuals for faunal groups) in the regionally most frequent production habitats (a), in the most frequent nonproduction habitats (b) and on total organism abundance per farm for the faunal groups (c).Xaxes are log-scaled to equalize distances on both sides of parity. Numbers onyaxis indicate the twelve regions shown inFig. 1a. Significant differences within regions (U-test) at 0.05 and 0.01 are indicated by * and **, respectively. Figure 4: Organic farming gains and losses to organism abundance in twelve regions. Organic farming gains/losses (OFG, ±s.d.) to organism abundance for the four taxonomic groups (cumulated cover for plants and number of individuals for faunal groups) in the regionally most frequent production habitats ( a ), in the most frequent nonproduction habitats ( b ) and on total organism abundance per farm for the faunal groups ( c ). X axes are log-scaled to equalize distances on both sides of parity. Numbers on y axis indicate the twelve regions shown in Fig. 1a . Significant differences within regions ( U -test) at 0.05 and 0.01 are indicated by * and **, respectively. Full size image Organic farming gains to species diversity at regional level There were considerable differences in species richness between regions for the four taxonomic groups. However, in the majority of regions, species accumulation curves from samples in organic and nonorganic farms had similar shapes ( Supplementary Figs 4–7 ). Extrapolated regional species numbers from these curves differed little between organic and nonorganic farms ( Supplementary Fig. 8a ) and the overall organic farming gain was +3.1% (NS). The organic farming effect on regional organism abundance was +12.4% (NS, Supplementary Fig. 8b ) and on regional species evenness −6.3% (NS, Supplementary Fig. 8c ). The evidence from 205 European and African farms suggests substantial organic farming gains to species richness of plants and bees in production habitats in intensive arable regions, which is in agreement with several other studies conducted at the field level [11] , [15] , [16] , [17] , [18] , [19] , [20] , [22] . Organic farming benefits to species richness in production fields increased with regional average nitrogen input, as well as with differences in nitrogen input between organic and nonorganic farms. This agrees with a recent meta-analysis [22] as well as with an investigation in wheat fields, which indicated that organic farming gains in biodiversity are proportional to losses in yield [21] . However, organic farm gains to species richness at the field level fade when observed at a greater spatial level, from a significant +10.5% overall taxa at the field level to a marginal +4.6% at the farm and +3.1% at the regional level. Our finding is in agreement with the few studies that compared organic and nonorganic practices at farm or landscape level and found weaker effects at higher levels of aggregation [12] , [19] . In contrast to earlier studies, we aimed at a comprehensive assessment of all habitats affected by farming activities, including nonproductive habitats, such as unpaved tracks or field margins. This allowed us to account for possible differences in habitat composition between farms, which are of crucial importance for biodiversity at farm level [28] , [33] , [34] , [35] . Species richness at the farm level is a combination of farming effects at the field level and the composition of farmland habitats on each farm. This interaction is exemplified by comparing data from Extremadura and Veneto. In Extremadura, organic and nonorganic olive groves (the production habitat) did not differ in species richness because in both farming systems, the primary management is harrowing to control weeds and reduce competition for soil water [36] . Herbicides are primarily used to control weed invasion from margins and reduce species richness in nonorganic nonproduction strips of grass and shrubs. Consequently, less species are found in nonorganic than in organic farms. In contrast, herbicide use in nonorganic vineyards in Veneto reduced floral species richness [37] , while the application of natural pesticides and organic weed control may have reduced richness of faunal groups in organic vineyards [38] . Similar habitat richness in all farms resulted in higher floral but lower faunal species richness on organic than nonorganic Venetian farms. Habitat composition was taken into account in the resampling procedure, which highlights a continuous decrease in the positive effects of organic farming on plant and bee species richness as more farm habitats are sampled. Such fading from field to farm may be explained by two processes: the regional pool of farmland species may be limited and simply attained faster on organic farms, or additional species in organic production habitats are ubiquitous, invading more easily from boundaries into fields and contribute little to the total species richness per farm. Ubiquity of species appears to be more likely than limited pools as the individual farms contained, on average, only 27% (±6.8% s.d.) of all plant species and 24% (±13.2%) of all bee species found in the region. We further calculated the occurrence of each plant and bee species relative to all samples in a region as a measure of species rarity, but did not find organic farming effects on species rarity. This suggests that the higher species richness in organic production fields is mostly due to common species, which contribute relatively little to total farm species richness because they are frequently found in other habitats of each farm. There was a striking correspondence between gains to species richness and organism abundance across all regions and taxonomic groups. Although this is not surprising and is a well-known property of species richness [25] , [30] , [39] , it shows that a higher abundance of individuals is likely the most important effect of organic farming on species richness. Hence, organic farming is not significantly increasing the number of species present in a given number of individuals but sustains a higher number of individuals in a given sampling unit. Investigating species diversity across multiple regions and taxonomic groups using standardized methodology also substantially complements our understanding of the effects of organic farming on biodiversity by showing where there are no significant effects. Most prominently, organic farming contributed little to habitat heterogeneity, which is of key importance for farmland biodiversity [28] , [33] , [34] , [35] . Organic and nonorganic farms did not differ in average habitat richness and thereby, in their potential to host exclusive species in any of the investigated regions. Organic farming effects on earthworm and spider richness and abundance were highly region-specific but marginal over all regions. Furthermore, we found significant gains to species evenness in plants in arable fields only, in contrast to a recent meta-analysis based on 81 studies [25] . This shows that any evaluation of farming effects on biodiversity requires critical consideration of the investigated taxonomic groups and geographical coverage [22] , [40] . Organic farming gains in the two investigated African regions were surprisingly small and did not differ from European regions. Interestingly, plant species richness in both regions tended to be lower in organic than in nonorganic production fields. Due to the costs of organic certification and market access, organic growers may invest more labour in weed control than some of their nonorganic counterparts [41] . In addition, inputs to agriculture are relatively low in both regions and, hence, differences between organic and nonorganic management are small [42] . Despite substantial variation between taxonomic groups and regions, the majority of the average effects of organic farming on species diversity demonstrate a positive tendency. This is true for most of the nonsignificant effects on species richness, abundance and evenness in productive fields and at farm and regional level. Hence, organic farming tends to sustain species diversity to a higher degree than nonorganic farming by allowing more individuals to survive in a given unit of agricultural habitat. We conclude that organic farming represents a step in the right direction toward preserving farmland biodiversity. Yet, the gains fade at the farm level due to the equilibrating effect of nonproduction habitats, which are similar in both farming systems. Therefore, land sharing by present-day organic farming alone is unlikely to halt the current global decline in farmland biodiversity [1] , [14] . Additional land-sparing measures that maintain and increase habitat diversity and quality, such as directed agri-environment schemes [6] , [18] , [27] , set-aside areas [29] , [34] and management contracts for habitats of rare species [7] are urgently needed. Implementation of these measures in organic farming guidelines [8] , [9] should be intensified to boost its performance in terms of promoting farmland biodiversity. Our study highlights that only by means of such targeted measures it is possible to accommodate the dual objectives of food production and biodiversity conservation on farmland. Study regions and farms Study regions were selected to reflect major organic farming types in Europe and Africa as well as to be spread across a large gradient of climatic conditions ( Table 1 ). To minimize farm selection bias, the regions needed to be as homogeneous as possible with respect to environmental conditions (soil, temperature and precipitation), while still containing a sufficient number of organic and nonorganic farms. Basic farm information was obtained from local sources ( Supplementary Table 1 ) and specific exclusion criteria were applied to all farms within each study region, for example, a minimum portion of area under arable cropping for farms in regions with mixed land use, a minimum farmed area, a particular livestock type or the cultivation of a particular crop. Hence, sampled farms were representative for a specific combination of region and agricultural types, for example, vine producers in Veneto, but not for all farms in a region. Organic farms were required to have been certified organic for at least 5 years before the study. No additional constraints were set on the nonorganic farms. Out of the eligible farms in each region, 8 to 10 organic and an equal number of nonorganic farms were selected at random ( Supplementary Table 1 ). If no agreement was provided by farmers, reserve random selections were used to complete the set. In the Hedmark region, the total number of farms studied was limited to 12 due to sampling time constraints caused by the short growing season and the complex habitat structure. In the entire Gelderland region, only three nonorganic horticultural farms within the study region agreed to participate in the study, in comparison with 11 organic farms. In Homokhatsag, only seven organic farms were available for investigation and in Obwalden, a nonorganic farmer ceased participation during the study. In Veneto, farms had to be selected from three separate vine areas because there were not enough organic farmers within one single area. In Wales and Hedmark, organic and nonorganic farms were selected in pairs because they were located along a geographical and intensity gradient that made it difficult to get an unbiased subset by random sampling. Detailed farm data and management information was gathered during structured interviews with farmers. Nitrogen input in kg N ha −1 included nitrogen from mineral and organic fertilizers as well as estimated N 2 fixation and was compared with national average nitrogen inputs in kg N ha −1 in 2008 (ref. 43) [43] . Counts of mechanical operations included field cultivation, pesticide applications, mowing, turning, bale making and loading. Counts of pesticide applications included natural pesticides. N input, mechanical operations and pesticide applications on fields were totalled and the area-weighted averages per farm were calculated. Gathering of management information in African countries involved more uncertainty than in Europe, especially in multiple cropping systems and the characterization of organic fertilizers. Hierarchical preferential sampling The entire area of each study farm was mapped according to the EBONE methodology, a standard habitat mapping procedure for the European scale [44] , [45] . This method is based on a generic system of habitat definitions, General Habitat Categories (GHCs). The habitat qualifiers, which characterize individual habitats with respect to their ecological features, include categories specifically related to farming areas. For our study, the method has been adapted with refined GHC definitions to deal with the specific characteristics of farm holdings. The most important adaptation was the division of the annual crop GHC into four subcategories, namely summer or winter-sown non-entomophilic annuals, entomophilic and/or bee-attracting annuals and perennials. In addition, the three dominant plant species were recorded and allowed for comparisons within the regionally most frequent crops. The first step in mapping was the assessment of the farm area, that is, all land managed by a farmer. In the second step, the area was mapped to either areal or linear elements. The minimum mappable area for an areal element was 400 m 2 , with minimum dimensions of 5 m × 80 m. If the width of an element was smaller than 5 m, it was recorded as a linear element with a minimum mappable length of 30 m. Third, based on life form and nonlife form categories, a GHC was assigned to every areal and linear element. A farm class (farmed and non-farmed land) and specific environmental and management qualifiers were attributed to all areal elements. The GHCs and qualifiers were chosen from a limited list using specific rules to avoid potential multiplicity of codes and mosaics, and to provide a lowest common denominator for linking data sets across study regions. The combination of GHCs and qualifiers allowed a specific separation of habitats with distinct species compositions (for example, grasslands of different management intensity), while still being general enough for comparison within regions. Across all 12 study regions, the habitat mapping yielded 167 distinct habitats on farmed land, with an average of 26 (range of 13–58) in each region and an average of 7.2 (1–15) per farm ( Supplementary Table 2 ). Out of all areal or linear elements of a specific farmed habitat on each farm, one plot was randomly selected. On the selected plots, the species of the four taxonomic groups were sampled in 2010 and 2011 using standardized protocols [46] . Species sampling Plant species in selected plots of areal habitats were recorded in squares of 10 m × 10 m, well away from the plot edges. In linear habitats, which were by definition less than 5 m wide, plant species were recorded in a rectangular strip of 1 m × 10 m. Earthworms were extracted at three random locations per plot in all regions except Monastir/Madhia, where they were completely absent. When soil was humid, 2 litres of a solution of allyl isothiocyanate, a commercially produced metabolite of glucosinolate, were poured into a metal frame (30 cm × 30 cm) twice at 5-min intervals [47] and earthworms appearing at the surface were collected. Thereafter, a soil core of 30 cm × 30 cm × 20 cm depth was excavated, and a single person hand-sorted the earthworms from the soil for a duration of 20 min. Spiders were caught with a vacuum shredder (Stihl SH 86-D, Andreas Stihl & Co., 64807 Dieburg, Germany) with a tapering gauze bag inserted into the intake nozzle [48] . On each of the three sampling dates, five subsamples were collected for 30 s within a sample ring of 0.357 m internal diameter haphazardly pre-placed on the target vegetation within each plot. Subsamples were immediately transferred to a cool-box. As a taxonomic catalogue of spiders is lacking in the Kayunga region, the region was not sampled for spiders. Bees were captured with a standard entomological aerial net along a transect of 100 m length and 2 m width during 15 min [49] , [50] , either identified in the field or immediately transferred into a kill jar. Domesticated bees were counted in the field but not captured. Each plot was surveyed three times during the growing season, but specific timing depended on local conditions. Metrics of species diversity Organism abundance and species richness at the field level was calculated by summing all individuals and species per plot, respectively. Species evenness was calculated as where a i is the log-transformed abundance of species i , ā is the mean of all a i and S is the total number of species [25] , [51] . Data points without or with only one sampled species were omitted from the evaluation of evenness, as no meaningful values could be calculated. Total species richness at the farm level was calculated by counting all species observed in all the sampled habitats on each farm. Abundance at the farm level was calculated by totalling all individuals in all the sampled habitats on each farm. Species richness of faunal groups was rarefied individual-based to the smaller value between two and the lowest number of individuals present in all the samples of one region using Hurlbert’s method [52] implemented in package vegan 2.0–10 in R 3.0.1 (ref 53 ). Presented values therefore still reflect differences in the frequency of plots where 0 and 1 individual was sampled. Total species richness at the regional level was calculated by extrapolating the species-area curves ( Supplementary Figs 4–7 ) using the jackknife method of first order [54] . Furthermore, moment-based species accumulation curves together with unconditional standard deviations [55] were calculated for all samples collected on organic and nonorganic fields in each region. Statistical analysis Differences between organic and nonorganic within individual regions were tested using Mann–Whitney U tests. Because interpreting the significances of these tests is not trivial in light of the numerous comparisons [56] , we relied on mixed-effects models for assessing the impact of organic farming. In these models, farming effects on each metric of species diversity ( S ) were calculated for each taxonomic group over all the 12 regions. For organism abundance and species richness, the data were ( S ij | β , b , x ) ~\n Poisson( μ ij ) from i =1, …, 205 farms in j =1, …, 12 regions. The model is: where β 0 is a fixed intercept, β 1 a fixed effect of farming treatment x 1 ij (organic versus nonorganic), β 2 is a fixed effect of the number of sampled habitats per farm x 2 ij , b 1 j are random intercepts for country j , and b 2 ij are random intercepts for farm ij . Random effects b 1 to b 2 are normally distributed with mean 0 and variance σ 2 . Random intercepts b 2 ij accommodate extra-Poisson variance due to over-dispersion [57] . The significance of term β 1 was calculated by log-likelihood ratio tests with one degree of freedom [58] , p. 83 . For species evenness, mixed-effects models analogous to equation (2) but with a Gaussian error structure were estimated. As the number of sampled habitats on each farm was not equal across farms, it was incorporated into the models for species richness and abundance at the farm level as a linear covariate x 2 ij [59] , p. 112 . The number of samples had no effect at the field level and was omitted from these models. Maximum-likelihood estimation was carried out in R 3.0.1 (ref. 53) [53] using package lme4 (Version 0.999999-2). The models over all four taxonomic groups are more complex and, hence, offer several possible structures of random effects. For each metric of species diversity, we started therefore with a complex structure of random effects (full model) and subsequently simplified it using sequential log-likelihood ratio tests [58] . The most parsimonious model was finally used for inference on the overall organic farming gain to species richness. For each evaluated measure of species richness and abundance ( S ), the data were species richness ( S kij | β , b , x ) ~\n Poisson( μ kij ) of k =1, …, 4 taxonomic groups from i =1,…, 205 farms in j =1,…, 12 regions. The full model is where β 0 is a fixed intercept, β 1 is a fixed effect of farming treatment x 1 ij (organic versus nonorganic), β 2 is a fixed effect of the number of sampled habitats x 2 ij in farm ij , and β 3 k is a fixed intercept for the taxonomic group k . The term b 1 j is a random intercept for country j , b 2 jk is a random intercept for the combination of country j and taxonomic group k , and b 3 ij is a random intercept for farm ij . The term b 4 ijk is a random intercept for observations of taxonomic group k in farm ij and accommodates extra-Poisson variance due to over-dispersion [57] . Random effects b 1 to b 4 are normally distributed with mean 0 and variance σ 2 . Term b 5 ij is a random effect of taxonomic group k within farm ij . To account for the nestedness of the observations of the four taxonomic groups within farm ij , b 5 ij is multivariate normal, with mean 0 and covariance matrix Σ. The most parsimonious models of both measurements of species richness and organism abundance at field level were full models without the fixed term β 2 and without random terms b 2 and b 3 .The most parsimonious model of species richness and organism abundance at farm level was the full model without random terms b 1 , b 3 and b 4 . Significance of term β 1 was calculated by a log-likelihood ratio test with one degree of freedom [59] . Calculation of organic farming gain/loss For individual regions and taxonomic groups, organic farming gains (OFGs) and losses were calculated as percent difference of organic farms (OFs) relative to nonorganic farms (NOFs) where is the mean in organic and nonorganic farms in each region. The standard deviation [60] of the OFG is where s.d. is the standard deviation and n is the number of observations in each group. Organic farming gains and losses across regions and taxonomic groups were calculated based on coefficients estimated from mixed-effect models (equations 2 and 3). At the population mean, the expected effect of organic farming is e β 0+ β 1 /e β 0 =e β 1 and hence Area-weighted random resampling To assess the diminishing of organic farming gains to species richness from field to farm, we resampled fields according to their proportion of total farm area. Specifically, we generated 100 random sequences of all sampled habitats per farm weighted by their areal proportion [61] , p. 111 . This resulted in random sequences of habitats predominantly starting with those habitats with high areal proportions. We then calculated the accumulation of species richness along each sequence and, based on the 100 realizations, the mean accumulation of species richness per farm. Finally, we fitted mixed-effects models for each taxonomic group at each number of sampled habitats using equation (2) and calculated organic farming gains using equation (6). How to cite this article: Schneider, M. K. et al. Gains to species diversity in organically farmed fields are not propagated at the farm level. Nat. Commun. 5:4151 doi: 10.1038/ncomms5151 (2014).